Identification of a human neonatal immune-metabolic network associated with bacterial infection Understanding how human neonates respond to infection remains incomplete. Here, a system-level investigation of neonatal systemic responses to infection shows a surprisingly strong but unbalanced homeostatic immune response; developing an elevated set-point of myeloid regulatory signalling and sugar-lipid metabolism with concomitant inhibition of lymphoid responses. Innate immune-negative feedback opposes innate immune activation while suppression of T-cell co-stimulation is coincident with selective upregulation of CD85 co-inhibitory pathways. By deriving modules of co-expressed RNAs, we identify a limited set of networks associated with bacterial infection that exhibit high levels of inter-patient variability. Whereas, by integrating immune and metabolic pathways, we infer a patient-invariant 52-gene-classifier that predicts bacterial infection with high accuracy using a new independent patient population. This is further shown to have predictive value in identifying infection in suspected cases with blood culture-negative tests. Our results lay the foundation for future translation of host pathways in advancing diagnostic, prognostic and therapeutic strategies for neonatal sepsis. Despite advances in neonatal care, infection remains a leading cause of morbidity and mortality in neonates worldwide. Although progress towards survival of children under the age of 5 years has been made as one of the Millennium Development Goals, neonatal morbidity and mortality remain a major issue in resource-rich and -poor settings [1] . Of 7.6 million deaths in children younger than 5 years in 2010, 64.0% (4.879 million) were attributable to infectious causes and 40.3% (3.072 million) occurred in neonates [1] . Up to 65% of extremely low-birth-weight infants develop presumed sepsis in the neonatal period [2] . Accordingly, there is a low threshold for clinical suspicion of infection in neonates, particularly as presentation varies greatly from very subtle signs to catastrophic collapse. Empirical antibiotics are widely used because of the lack of reliably sensitive tests and the potential life-threatening consequences of delayed treatment of infection. This exposes many infants without infection to broad-spectrum antibiotics. Clinical investigation of neonates is problematical and our understanding of neonatal sepsis is hampered by a lack of appropriate animal models and species-specific differences in response to infection. Neonates are more susceptible to infection than older individuals, however, neonatal immunity is not well characterized [3] . Moreover, host responses are known to play a significant role in the pathophysiology of sepsis; yet our understanding of how humans respond at the systemic pathway level to infection in early life is not known. Systems investigations using genomics, in particular, are increasingly used to examine host–pathogen interactions in an unbiased manner [4] , [5] , [6] . Changes in host gene expression may occur pre-symptomatically in response to infection in any part of the body, with the continuous interaction between blood and tissue allowing blood cells to act as internal biosensors for the changes [6] , [7] . Studies have examined transcription profiles of blood from adults and children with infection, but data from infected neonates are lacking [4] , [8] , [9] , [10] , [11] , [12] . However, a limited number of host markers at the protein level have been investigated in neonates [13] , [14] , [15] , [16] , [17] . It is likely that neonatal transcriptional responses differ from other age groups because neonates are developmentally immature and may be encountering infection for the first time. Towards applying a systematic system-level investigation, we previously assessed variability and statistical power of measuring neonatal whole blood RNA [18] . These studies lent support to the notion of using whole blood rather than peripheral blood mononuclear cell profiling for a more full picture of the host response. Furthermore, before extensive clinical investigations we developed a high-performance computing model for host RNA classification. These simulations demonstrated that as few as 24 whole blood RNA markers (comprising biological pathways) would be sufficient for predicting infection [19] . These studies and those published by others in older infected individuals support the approach of using host whole blood RNA to systematically identify the pathway biology underlying the pathogenesis of neonatal infection. In this study, we characterize the pathway biology underlying neonatal sepsis at the first clinical signs of infection. We derive and validate a panel of pathway biomarkers that are further clinically evaluated for potential future translation in stratifying neonatal infection. Vigorous systemic host RNA perturbation in neonatal infection First, we assessed the magnitude and extent of variability of gene expression using the training set and one virally infected case. In these analyses, 23,342 probes gave detectable signal for one or more samples. Of these, 10,206 showed a coefficient of variation of >0.1 across all 63 samples. A principal components analysis of patient samples based on these 10,206 probes and agglomerative unsupervised clustering of normalized unfiltered data revealed a separation into control and infected groups ( Fig. 1a and Supplementary Fig. 1 ). The single exception was the virally infected case and was excluded from later analyses. 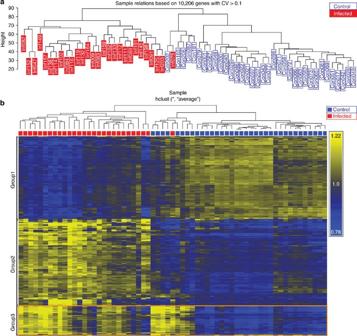Figure 1: Hierarchical clustering of infected and control patient samples. (a) Results from unsupervised analysis of normalized data before statistical testing. At this stage, the condition of whether the samples were infected or not had not been included in the analysis. Control, blue; infected, red. (b) Heat map showing hierarchical clustering of infant samples based on the 824 probes that were statistically differentially expressed between infected and control groups (using eBayes with Benjamini-Hochberg correctionadj.P≤0.01, absolute fold change ≥2). Hierarchical clustering was based on Euclidean distance. Three clusters of genes are labelled (1–3). Group 3 genes (highlighted with an orange box) were excluded from the further analysis for derivation of a classifier of neonatal bacterial infection because of no clear separation between infected and controls. Control, blue; infected, red. Figure 1: Hierarchical clustering of infected and control patient samples. ( a ) Results from unsupervised analysis of normalized data before statistical testing. At this stage, the condition of whether the samples were infected or not had not been included in the analysis. Control, blue; infected, red. ( b ) Heat map showing hierarchical clustering of infant samples based on the 824 probes that were statistically differentially expressed between infected and control groups (using eBayes with Benjamini-Hochberg correction adj.P ≤0.01, absolute fold change ≥2). Hierarchical clustering was based on Euclidean distance. Three clusters of genes are labelled (1–3). Group 3 genes (highlighted with an orange box) were excluded from the further analysis for derivation of a classifier of neonatal bacterial infection because of no clear separation between infected and controls. Control, blue; infected, red. Full size image Statistical testing further underscored the large-scale demarcation of response, revealing 8,242 significantly differentially expressed probes ( adj.P ≤0.01) with adjusted P values as low as 10 −23 . By applying statistical and quantitative cutoffs ( adj.P ≤0·01, absolute fold change ≥2) this was reduced to 824 and accordingly represents a global signature of infection for a naïve neonatal immune system. Euclidean distance-based clustering of the 824 differentially expressed probes ( Fig. 1b and Supplementary Data set 1 , worksheet 1) revealed upregulated (yellow) and downregulated (blue) genes in infection, demarcated by three groups: group 1 representing downregulated; group 2 those upregulated; whereas group 3 showing no clear separation between infected and controls. Many of the 118 probes in group 3 encode functions related to blood development ( Supplementary Fig. 2i,j ) and were excluded from subsequent analyses. Pathway biology responses to infection To identify the most highly active set of pathways associated with infection, we applied additional filtering to groups 1 and 2 using more stringent cutoffs ( adj.P ≤10 −5 , fold change ≥4). Analysis of the resulting 52 genes revealed sub-networks (termed ‘dual-network’), for upregulated and downregulated expression. The dual-network shows a uniformly clear signal separation into activated (yellow) and suppressed (blue) genes in infected cases ( Fig. 2a ) and consists of three functional pathway classes of innate and adaptive immunity and unexpectedly metabolic pathways for sugar and lipid metabolism ( Fig. 2b–e and Supplementary Fig. 3 ). Overall, these results show a vigorous systemic host RNA network perturbation upon bacterial infection. 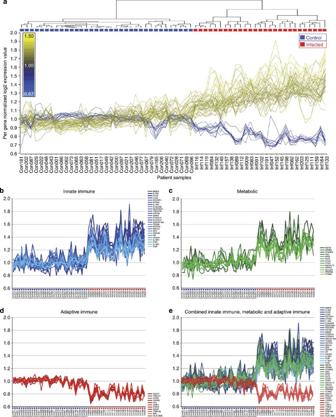Figure 2: 52-Gene dual-network classifier of neonatal bacterial infection comprised of innate, metabolic and adaptive immune pathways. (a) Line graph of per gene normalized expression values using the 52-gene dual-network classifier of neonatal bacterial infection with sample order determined using hierarchical clustering based on Euclidean distance. Line graphs of per gene normalized expression values using genes associated with (b) innate immune, (c) metabolic, (d) adaptive immune and (e) combination of all three pathways present in the 52-gene dual-network classifier of neonatal bacterial infection. Control, blue; bacterial infected, red. Figure 2: 52-Gene dual-network classifier of neonatal bacterial infection comprised of innate, metabolic and adaptive immune pathways. ( a ) Line graph of per gene normalized expression values using the 52-gene dual-network classifier of neonatal bacterial infection with sample order determined using hierarchical clustering based on Euclidean distance. Line graphs of per gene normalized expression values using genes associated with ( b ) innate immune, ( c ) metabolic, ( d ) adaptive immune and ( e ) combination of all three pathways present in the 52-gene dual-network classifier of neonatal bacterial infection. Control, blue; bacterial infected, red. Full size image Immune signalling pathway To interrogate signalling pathways in groups 1 and 2, we performed hypergeometric tests using the Ingenuity Pathways Analysis (IPA) database (http:// www.ingenuity.com ), developing eight highly connected networks of functionally related genes ( Supplementary Fig. 2a–h ). Group 1 mapped to antigen processing and presentation via major histocompatibility complex II, lymphocyte differentiation, T-cell activation and T-cell receptor (TCR) signalling. Group 2 mapped to innate immune processes including Toll-like receptor (TLR), chemokine, interleukin (IL)-6, IL-1β and Janus kinase-Signal Transducer and Activator of Transcription (JAK-STAT) signalling, platelet activation and apoptosis. It is noteworthy that interferon (IFN)-γ, although expressed in all patient samples, is not differentially activated ( Fig. 3a,b ). Although this is consistent with the reduction in levels of expression of genes of the adaptive immune system ( Fig. 3a ), the IFNγ regulated gene CXCL10, showing a good correlation with STAT1 in infected cases ( r= 0.8) but not in controls ( r =0.3; Supplementary Fig. 4 ). 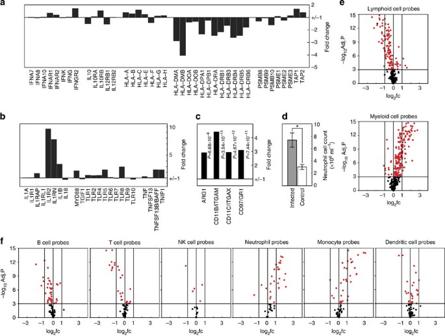Figure 3: Differential adaptive and innate immune responses to neonatal infection. (a) Fold change in expression of adaptive immune response genes following neonatal infection. (b) Fold change in expression of innate immune response genes following neonatal infection. (c) Fold change in expression of genes associated with myeloid-derived suppressor cells following neonatal infection. Significance is indicated by adjustedP-values for fold change of each probe (using eBayes with Benjamini-Hochberg correction). (d) Neutrophil cell counts from control and infected patients. Neutrophil cell counts were examined in control (n=12) and infected (n=28) patients and are expressed as numbers × 106cells per ml of blood with the plot presenting median values±median absolute deviation. Significance testing between conditions was performed using a one-way analysis of variance test, * indicates significance atP<0.0005. (e,f) Cell type enrichment analysis. Volcano plots of expression profiles associated with particular blood cell types and classes. Gene lists used to perform this analysis are detailed inSupplementary Data set 2. Log2fold change is on thexaxis and –log2adjustedPvalue on theyaxis (using eBayes with Benjamini–Hochberg correction). (e) Expression profiles for lymphoid and myeloid cells. (f) Expression profiles for B, T, NK cells, neutrophils, monocytes and dendritic cells. Significantly differentially expressed probes (withadj.P≤0.01) are shown in red. Figure 3: Differential adaptive and innate immune responses to neonatal infection. ( a ) Fold change in expression of adaptive immune response genes following neonatal infection. ( b ) Fold change in expression of innate immune response genes following neonatal infection. ( c ) Fold change in expression of genes associated with myeloid-derived suppressor cells following neonatal infection. Significance is indicated by adjusted P -values for fold change of each probe (using eBayes with Benjamini-Hochberg correction). ( d ) Neutrophil cell counts from control and infected patients. Neutrophil cell counts were examined in control ( n =12) and infected ( n =28) patients and are expressed as numbers × 10 6 cells per ml of blood with the plot presenting median values±median absolute deviation. Significance testing between conditions was performed using a one-way analysis of variance test, * indicates significance at P <0.0005. ( e , f ) Cell type enrichment analysis. Volcano plots of expression profiles associated with particular blood cell types and classes. Gene lists used to perform this analysis are detailed in Supplementary Data set 2 . Log 2 fold change is on the x axis and –log 2 adjusted P value on the y axis (using eBayes with Benjamini–Hochberg correction). ( e ) Expression profiles for lymphoid and myeloid cells. ( f ) Expression profiles for B, T, NK cells, neutrophils, monocytes and dendritic cells. Significantly differentially expressed probes (with adj.P ≤0.01) are shown in red. Full size image IPA analysis of the 52-gene dual-network confirmed the three pathways of innate, adaptive and metabolic. The upregulated sub-network forms a myeloid innate immune and metabolic signature anchored around matrix metallopeptidase 9 (MMP9) and lipocalin 2 (LCN2) associated with macrophage activation and lipid metabolism ( Fig. 2b ; Supplementary Fig. 3a ). Other metabolic genes include the free fatty acid receptor 2 (FFAR2/GPR43) that links short chain fatty acids, neutrophils and gut–microbiota interactions as well as glycolytic and energy metabolism ( Fig. 2c ; Supplementary Fig. 3a ). The downregulated pathway comprises lymphoid markers of adaptive immunity centred on the TCR/CD3 complex and associated TCR signalling pathways ( Fig. 2d ; Supplementary Fig. 3b ). Taken together, this analysis provides, for the first time, a link between metabolic and inflammatory processes in neonatal sepsis ( Fig. 2e ). Immune inhibitory signalling Notably, upregulation of inhibitory signalling pathways is observed. The decoy receptor for IL-1β (IL1R2) and the IL-1 receptor antagonist (IL1RN; Fig. 3b ) systemically counteract the inflammatory response, and is concurrent with a broad cell intrinsic inhibitory response. Cell intrinsic repressors include A20, IκBα, TOLLIP, TRAFD1, TRAIL-R3 (TNFRSF10C), IRAK-M, SOCS1 and SOCS3 that counter regulate the NF-κB, TLR, MYD88, IRAK and JAK-STAT signalling pathways, respectively ( Supplementary Fig. 5 ). These counter regulatory pathways affect the set-point in immune-homeostatic control (defined here as the level at which the innate immune system activates the adaptive response) that is governed by the net balance between inhibitory and stimulatory responses. Accordingly, although a significant number of infected infants show elevated CD163 macrophage-activation marker expression ( adj.P ≤10 −6 ), they also exhibit increased co-inhibitory ligands such as PD-L1 (CD274) that impedes T-cell proliferation and cytokine production. Moreover, genes associated with myeloid-derived suppressor cells are elevated (CD11B, CD97) including increased ARG1 that marks a potent anti-inflammatory phenotype ( Fig. 3c ). In relation to elevated ARG1, the CD71 erythroid cell marker was also upregulated ( Supplementary Fig. 5 ) and in neonates contributes towards the suppression of immune cell activation [20] . A corollary of the stimulatory and inhibitory signalling pathways is their likely impact on functional changes in immune cell compartments. Changes in immune cell compartment To investigate cellular compartments, we used markers of specific blood cell lineages [21] ( Supplementary Data set 2 ) to model cell-type-specific modules of RNA expression. An increased level of myeloid cells, especially monocytes and neutrophils, is inferred in infected samples ( Fig. 3e,f ; Table 1 ), which was validated by a significantly increased neutrophil cell count ( Fig. 3d ). Conversely, expression modules for lymphoid cells, particularly B and T cells were lower ( Fig. 3e,f ). A significant difference is not detected for either dendritic or natural killer cells ( Table 1 ). We conclude that in sepsis the heightened innate immune cellular response is driven by monocytes/macrophages and neutrophils and is counter-balanced by inhibitory pathways resulting in a net suppression of the adaptive immune arm, especially associated with the T-cell compartment. Table 1 Cell type enrichment analysis. Full size table Regulatory nodes To gain insight into the underlying regulatory nodes, we used the InnateDB resource [22] filtered for a high-confidence manually annotated data set of approximately 2,500 human molecular interactions. Analysis of direct interactions between group 2 genes ( Fig. 4a left) revealed those genes (represented as ‘nodes’ in the network) that are highly connected through direct physical or biochemical interactions (termed ‘hubs’) or which have many network shortest paths passing through them (termed ‘bottlenecks’) that mark potential key regulatory points in the network. The 20 major hubs were identified, of which the top four included immune regulatory factors STAT1, STAT3 and C/EBP-B, and the TNFR1 receptor ( Fig. 4a middle). The level of innate immune response triggering reflects the set-point for homeostatic immune regulation, and the activity of these nodes points to a heightened set point. The network was further analysed to identify ‘active sub-networks’ via the identification of high scoring sub-networks using a search algorithm based on simulated annealing [23] . The top-ranked upregulated sub-network ( Fig. 4a right), consisted of 81 nodes and 176 edges and was enriched in genes involved in Formation of Platelet plug , Fc gamma R-mediated phagocytosis , Platelet Activation , Hemostasis , Integrin signalling and chemokine signalling pathways . 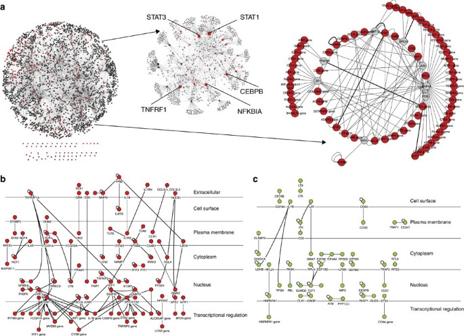Figure 4: Networks of experimentally supported direct molecular interactions between genes differentially regulated in neonatal sepsis. (a) Network relationships derived from InnateDB were visualized with Cytoscape. (Left) Network of direct molecular interactions between genes upregulated in neonatal sepsis patients (shown in red), their encoded products and all other interacting molecules. Inclusion of non-differentially expressed interacting partners (shown in grey) in this network allows potential identification of important regulatory nodes (genes/proteins) not evident from microarray data alone (for example, constitutively expressed nodes/nodes expressed at a time point not sampled in the study). (Middle) The top five hub nodes identified by Degree algorithm of cytoHubba plugin are labelled. Node sizes are defined by the node degree— the larger the node size the higher the degree. Nodes encoded by upregulated genes are shown in red, the top 20 hubs identified by this analysis were STAT1, STAT3, NFKBIA, TNFRF1, CEBPB, SPI1, LYN, BCL6, PRKCD, HCK, MYD88, HSPA1B, UBA1, CEBPD, JUNB, IRF7, TNFAIP3, CTNNA1, ETS2 and GNAI2. (Right) The top-scoring upregulated sub-network identified by jActiveModules plugin. Nodes representing upregulated RNA signals are shown in red; non-differentially expressed genes in grey. (b) Network of molecular interactions directly between genes upregulated in neonatal sepsis patients visualized with the Cerebral v.2 plugin. Nodes encoded by upregulated genes are shown in red; non-differentially expressed interactions partners are not shown. (c) Network of molecular interactions directly between genes downregulated in neonatal sepsis patients visualized with the Cerebral v.2 plugin. Nodes encoded by downregulated genes are shown in green; non-differentially expressed interaction partners are not shown. Figure 4: Networks of experimentally supported direct molecular interactions between genes differentially regulated in neonatal sepsis. ( a ) Network relationships derived from InnateDB were visualized with Cytoscape. (Left) Network of direct molecular interactions between genes upregulated in neonatal sepsis patients (shown in red), their encoded products and all other interacting molecules. Inclusion of non-differentially expressed interacting partners (shown in grey) in this network allows potential identification of important regulatory nodes (genes/proteins) not evident from microarray data alone (for example, constitutively expressed nodes/nodes expressed at a time point not sampled in the study). (Middle) The top five hub nodes identified by Degree algorithm of cytoHubba plugin are labelled. Node sizes are defined by the node degree— the larger the node size the higher the degree. Nodes encoded by upregulated genes are shown in red, the top 20 hubs identified by this analysis were STAT1, STAT3, NFKBIA, TNFRF1, CEBPB, SPI1, LYN, BCL6, PRKCD, HCK, MYD88, HSPA1B, UBA1, CEBPD, JUNB, IRF7, TNFAIP3, CTNNA1, ETS2 and GNAI2. (Right) The top-scoring upregulated sub-network identified by jActiveModules plugin. Nodes representing upregulated RNA signals are shown in red; non-differentially expressed genes in grey. ( b ) Network of molecular interactions directly between genes upregulated in neonatal sepsis patients visualized with the Cerebral v.2 plugin. Nodes encoded by upregulated genes are shown in red; non-differentially expressed interactions partners are not shown. ( c ) Network of molecular interactions directly between genes downregulated in neonatal sepsis patients visualized with the Cerebral v.2 plugin. Nodes encoded by downregulated genes are shown in green; non-differentially expressed interaction partners are not shown. Full size image An investigation of the regulatory interactions directly between nodes ( Fig. 4b ) showed a major connected component consisting of proteins involved in TLR (TLR5, TLR8, MYD88, IRAK3) and TNF signalling (among other pathways) leading to the transcriptional activation of a range of genes via a panel of transcription factors, including BCL6, CEBPB, CEBPD, ETS2, IRF7, JUNB, SPI1, STAT1 and STAT3. Minor components in the network consisted of genes involved in platelet activation (GNAI2, PPBP) and chemokine/cytokine signalling (GNAI2, IL8RA, IL8RB, PPBP) and involved in Fc-gamma R-mediated phagocytosis (DNM2, FCGR1A, FCGR2A, HCK, LYN). Next, we investigated interactions between downregulated nodes and all their interaction partners. The top 20 hubs in the downregulated network were identified and included the ETS1 transcription factor, several proteins involved in translation (EIF3E, EIF4A2, RPLP1, TUT1), two involved in cell cycle regulation (ATM, RBL2) and the cytokine receptor, IL7R. Many of these nodes were also identified as network bottlenecks. The top three differentially expressed sub-networks consisted of a network enriched in genes involved in translation, the HNF4A transcriptional module and a network enriched in components of TCR signalling ( Fig. 4c ). Taken together, we conclude that the overriding pathophysiological signal associated with neonatal infection is one of the increased innate immune metabolic responses with an unbalanced homeostatic regulation of adaptive immunity. The specific and intense activation of innate immune signalling, moderated via inhibitory pathways is consistent with the notion of an elevated set point in neonates in comparison with adults for guiding a suppressed adaptive immune response [24] . Metabolic pathway biology and immune homeostasis Unexpectedly, we found marked transcriptional changes in specific metabolic pathways, principally associated with glucose, energy and cholesterol metabolism ( Supplementary Fig. 5 ). For cholesterol biosynthesis and homeostasis, we find significant alterations in SQLE, IDI1, DHCR7, SCAP, INSIG2, NR1H2, ABCA1, LDLR and LDLRAP1 ( Supplementary Fig. 5 ). In the case of the glycolysis pathway, three key regulatory nodes of the pathway form part of the 52-gene dual-network ( Fig. 2c ). These are increased levels of the glucose transporter GLUT3 (SLC2A3), PFKFB3 (6-phophofructo-2-kinase) that activates the glycolytic flux under hypoxic conditions and HK3 a hexokinase that phosphorylates glucose to produce glucose-6-phosphate, the first rate-limiting step in glucose metabolism; and is indicative of changes in the tricarboxylic acid cycle. Another member of the dual-network involved in regulating lipid and glucose metabolism is lipocalin 2 (LCN2) [25] , [26] , which also plays a role in the innate immune response to bacterial infection by sequestering iron [27] , [28] , [29] , [30] . Other metabolic players of the dual-network include B4GALT5 that is responsible for synthesis of complex N-linked oligosaccharides for glycoproteins and glycolipids; and GYG1 that forms an oligosaccharide primer substrate for glycogen synthase. These metabolic processes are likely to be linked to the innate immune response. In support, analysis of the promoters of the metabolic sub-network identified 11 out of 13 genes containing binding sites for the myeloid-specific transcription factor PU.1 (SPI1), which is also part of the dual-network ( Supplementary Table 1 ). A crucial contribution to coupling homeostasis of host metabolism and the immune system is the microbial colonization of the intestine at birth. Here homeostatic regulatory pathways involve interactions between immune cells and metabolic products (primarily small chain fatty acids such as butyrate) of microbiota fermentation, which influences the set point for an immune response. In this connection, the free fatty acid receptor 2 (FFAR2/GPR43) plays a key role in linking the metabolic activity of the gut microbiota with body energy metabolism and immune activity and is an immune metabolic node within the dual-network. Systemically, FFAR2 is primarily expressed on neutrophils and granulocytes and a positive correlation between FFAR2 levels and the number of neutrophils in the control group is observable ( r =0.7), but this correlation is lost in bacterial infection cases ( r =0.2). This indicates that FFAR2 upregulation in sepsis is not due to increased neutrophil numbers but is suggestive of an immune-mediated upregulated response ( Fig. 5a ). STAT3 is one of the key immune-regulated hubs in sepsis ( Fig. 4a middle) and the FFAR 2 promoter has a predicted STAT3-binding site (Fisher score 0.9). In agreement, we find FFAR2 has a strong correlation with the levels of STAT3 in neonatal sepsis patients ( r =0.8) but not in the controls ( r =0.3; Fig. 5b ). In contrast, correlation between FFAR2 levels and FCN1 in either controls ( r =0.1) or infected group ( r =0.1) is low ( Fig. 5c ). M-ficolin (FCN1) encodes a collagen-type (C-type) lectin protein secreted by macrophages that binds FFAR2 on plasma membranes acting as part of the host innate immune activation pathway. Thus, rather than the host factor FCN1, microbial short-chain fatty acid metabolites derived from the gut microbiota such as butyrate likely act as the cognate ligands for FFAR2 on neutrophils, which functionally tunes the peripheral immune system [31] , [32] . These results will require further investigation but are consistent with the emerging view that the metabolic activity of the neonatal microbiota may contribute to control the systemic threshold of activation of innate and adaptive immune cells. 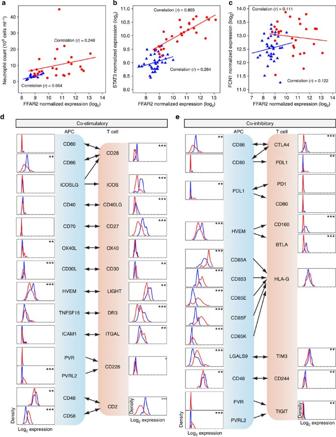Figure 5: Immune metabolic regulatory pathways. (a–c) Correlation analysis of FFAR2 gene expression with (a) neutrophil count, (b) STAT3 and (c) FCN1 (m-Ficolin) gene expression. Expression in control (blue) and bacterial infection (red) samples are shown. (d,e) Analysis of gene expression in molecules associated with T cell and antigen-presenting cell co-stimulatory (d) and co-inhibitory (e) interactions. Line graphs display gene expression as probability density plots for control (blue) and bacterial infection (red) samples. Graphs marked with asterisks indicate that the mean expression difference between the two study groups is statistically significant (using eBayes with Benjamini–Hochberg correction *P≤0.05, **P≤0.01, ***P≤0.001). Figure 5: Immune metabolic regulatory pathways. ( a – c ) Correlation analysis of FFAR2 gene expression with ( a ) neutrophil count, ( b ) STAT3 and ( c ) FCN1 (m-Ficolin) gene expression. Expression in control (blue) and bacterial infection (red) samples are shown. ( d , e ) Analysis of gene expression in molecules associated with T cell and antigen-presenting cell co-stimulatory ( d ) and co-inhibitory ( e ) interactions. Line graphs display gene expression as probability density plots for control (blue) and bacterial infection (red) samples. Graphs marked with asterisks indicate that the mean expression difference between the two study groups is statistically significant (using eBayes with Benjamini–Hochberg correction * P ≤0.05, ** P ≤0.01, *** P ≤0.001). Full size image The activity of immunosuppressive CD71 + erythroid cells has been implicated in suppressing host defence against infection in neonates [20] . Although expressed on a variety of blood cells, it is upregulated in sepsis but in only a small number of cases ( Supplementary Fig. 5 ) and is insufficient alone to explain the hypo-responsiveness of the adaptive arm. Homeostatic co-signal regulatory control The interaction between myeloid antigen-presenting cells and lymphoid T cells, serve as the immune control centre integrating homeostatic regulatory signals that govern the adaptive effector arm. Interaction of antigen–HLA complexes in T-cell activation requires two signals, TCR signalling and co-signal regulation. Moreover, naïve T cells are strongly dependent on co-signalling, which plays a vital role in either promoting or inhibiting T-cell activation. For the first TCR signal, expression of HLA class II is significantly downregulated in our sepsis cases ( Fig. 3a ). For the co-signal, CD80/CD86/CD28 interactions form the strongest co-stimulatory pathway and CD28-deficient cells fail to proliferate. In our neonatal sepsis cases, we find the differential gene expression for this pathway is dramatically diminished as well as expression levels of ICOS, CD27, LIGHT and CD2 ( Fig. 5d ). Although there was a small number of infected cases that showed increased TNFSF15, ICAM1, LFA-1 and 3 expression levels, the notably marked downregulation of CD3, LIGHT and CD2 was indicative of a suppression of T-cell priming that plays a role in the transition from quiescent to activated states ( Fig. 5d and Supplementary Fig. 5 ). In the case of co-inhibitory pathways, a highly specific and selective differential gene expression response was observed for the inhibitory receptor Ig-like transcripts (CD85A, CD85D and CD85K) [33] , [34] , [35] , [36] and potential dual co-inhibitory and co-stimulatory CD85E and CD85F transcripts ( Fig. 5e ). The increased expression of these receptors, in particular CD85K, converts T cells into suppressive cells [36] . Thus, examination of the complex co-signalling regulatory system reveals a highly focused and selective response in neonatal sepsis. Although these responses may be dynamically varied at the time of sampling, they clearly show quite a remarkably restricted and specific pattern. These negative regulatory pathways are suggestive of a significant new mechanism in neonates for contributing to suppression of the adaptive arm. Heterogeneity of infection-specific network responses We anticipate that individuals will have different responses. To examine this, we applied a data-driven approach for determining networks of co-expressed RNAs that are exclusive to infected infants. Modules were derived from the linear dependence of the 824 statistically significant gene probes and used a Markov Cluster Algorithm implemented in the BioLayout tool [37] for revealing correlated probes among patient samples. This type of analysis is highly subjective as clustering parameters are chosen visually by discerning discrete clusters termed ‘cliques’ and these will vary greatly in size and degree of connectivity dependent on the parameter chosen. Nevertheless, this approach is useful for exploring data-driven assignment of co-regulated genes for infected cases. 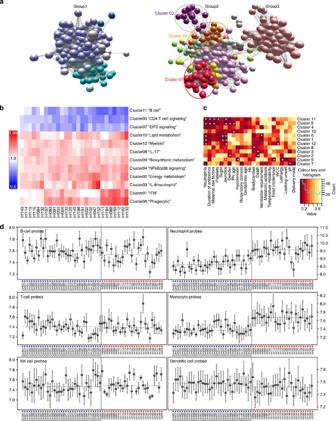Figure 6: Network analysis of patient-specific response to infection. (a) Patient-specific expression profiles. Networks of 824 statistically differentially expressed probes (using eBayes with Benjamini–Hochberg correctionadj.P≤0.01, fold change ≥2) visualized using BioLayout Express 3D. Three groups of genes are identified, which correspond to those identified by hierarchical clustering inFig. 1b. Co-expressed genes within networks were then defined with a Pearson correlationr=0.78 and by applying a Markov clustering (MCL) inflation value of 4 and pre-inflation value of 3 and are shown as coloured clusters (for example, Cluster 01 and so on). (b) Twelve MCL clusters of genes are displayed for bacterial infected patients to show patient-specific responses. Average expression values of MCL clusters were calculated from per gene normalized against mean of control samples and ordered by Euclidean distance. Full expression profiles of these clusters can be seen inSupplementary Fig. 6. (c) Twelve gene expression clusters showing heterogeneity within the group of infected neonates were tested for association with clinical parameters. For each infected neonate and cluster, median gene expression was calculated and tested for statistical association with each of the clinical parameters (seeSupplementary Data set 4). Wilcoxon rank sum tests were used to test association with binary clinical parameters, Spearman rank correlation tests were used to test association with continuous clinical parameters (sugar, neutrophil count, postnatal age, platelets, duration on antibiotics, pH, white cell count (WCC), hemoglobin (Hb), gestational age). The colour scale represents thePvalue estimate and asterisks identify Wilcoxon rank sum or Spearman rank correlation significant test outcome atP≤0.05. (d) Cell type enrichment analysis performed at an individual patient level shows patient-specific responses. Median signal levels for cell type-specific gene lists as detailed inSupplementary Data set 2are plotted (±median absolute deviation) for B, T, NK cells, neutrophil, monocyte and dendritic cells. Control, blue; bacterial infected, red. Figure 6a,b shows the developed modules of co-expressed genes using parameter cutoffs of Pearson correlation r =0.78 and Markov Cluster Algorithm inflation value of 4 and pre-inflation value of 3. In this analysis, 12 discernibly different modules are associated with infection and post-hoc pathway analysis shows each corresponding to a defined biological process ( Fig. 6b , Supplementary Fig. 6 and Supplementary Data set 1 , worksheet 2) and agrees with the pathway biology investigations described in the previous section. These modules clearly reveal an underlying heterogeneity in terms of an individual patient’s response to infection. For example, cluster 01 defines a specific type I IFN sub-network (and we note that the type II IFN responsive gene CXCL10 is a member of this network, suggesting redundant cross-talk between type I and II signalling). Type I IFN signalling can in some cases be detrimental for individuals with bacterial infection [38] . In individuals exhibiting cluster 01, we cannot rule out that those patients showing a type I IFN response may also be virally infected. Statistical association of the 12 networks with 23 clinical parameters was investigated ( Fig. 6c ). Sugar levels were associated with clusters 01 and 06. The association with cluster 01 is not obvious and may be indicative of STAT regulation of glycolysis, whereas cluster 06 consists of members associated with glycerol uptake and metabolism. The most common association was with neutrophils and clusters 01, 05, 06, 11 and 12, whereas none of the clusters are associated with gestational age. It should be considered that the overall sample size for these associations is small and will require further validation studies. Figure 6: Network analysis of patient-specific response to infection. ( a ) Patient-specific expression profiles. Networks of 824 statistically differentially expressed probes (using eBayes with Benjamini–Hochberg correction adj.P ≤0.01, fold change ≥2) visualized using BioLayout Express 3D. Three groups of genes are identified, which correspond to those identified by hierarchical clustering in Fig. 1b . Co-expressed genes within networks were then defined with a Pearson correlation r =0.78 and by applying a Markov clustering (MCL) inflation value of 4 and pre-inflation value of 3 and are shown as coloured clusters (for example, Cluster 01 and so on). ( b ) Twelve MCL clusters of genes are displayed for bacterial infected patients to show patient-specific responses. Average expression values of MCL clusters were calculated from per gene normalized against mean of control samples and ordered by Euclidean distance. Full expression profiles of these clusters can be seen in Supplementary Fig. 6 . ( c ) Twelve gene expression clusters showing heterogeneity within the group of infected neonates were tested for association with clinical parameters. For each infected neonate and cluster, median gene expression was calculated and tested for statistical association with each of the clinical parameters (see Supplementary Data set 4 ). Wilcoxon rank sum tests were used to test association with binary clinical parameters, Spearman rank correlation tests were used to test association with continuous clinical parameters (sugar, neutrophil count, postnatal age, platelets, duration on antibiotics, pH, white cell count (WCC), hemoglobin (Hb), gestational age). The colour scale represents the P value estimate and asterisks identify Wilcoxon rank sum or Spearman rank correlation significant test outcome at P ≤0.05. ( d ) Cell type enrichment analysis performed at an individual patient level shows patient-specific responses. Median signal levels for cell type-specific gene lists as detailed in Supplementary Data set 2 are plotted (±median absolute deviation) for B, T, NK cells, neutrophil, monocyte and dendritic cells. Control, blue; bacterial infected, red. Full size image The inter-patient variability of the modules is both qualitatively and quantitatively high and severely limits their use for a host-directed infection signal. Further heterogeneity is observed in inter-patient responses for immune cell compartments ( Fig. 6d ). For instance, although most sepsis cases show high levels of neutrophil markers, a small subset have levels commensurate with neutropenia. Thus, an examination of the cellular compartments is also insufficiently uniform. By contrast, the 52-gene dual-network identified using statistical and pathway information alone ( Fig. 2a ) is uniformly representative of a patient-invariant infection response. Moreover, there are no significant confounding associations with any of the 23 clinical parameters tested for the 52-gene dual-network. 52-Gene dual-network accurately predicts neonatal infection To test whether the 52-gene dual-network has predictive value, we applied four distinct machine-learning algorithms: random forest, support vector machine, k-nearest neighbour and receiver operator characteristics (ROC) for classification. Algorithm performance was assessed, with respect to node performance, by estimating the generalization error (measuring how well a learning-algorithm performs in new and unseen data) using a replicated leave-one-out cross-validation (LOOCV) approach. We replicated the cross-validation algorithm 100 times averaging out any variation in error estimates resulting from randomness while splitting the data set into training and test sets at each step. 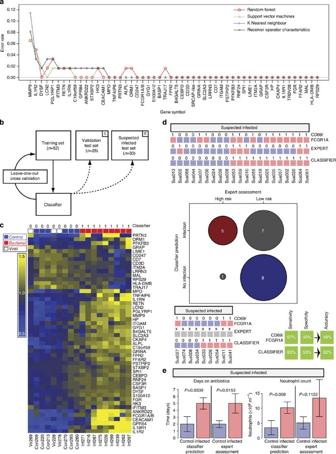Figure 7: Validation of the 52-gene dual-network classifier. (a) Members of the network as a classifier of neonatal infection using leave-one-out cross-validation analysis using four independent machine-learning algorithms (red circle, random forest; green triangle, support vector machines; blue+, K nearest neighbour and black x, receiver operator characteristics). (b) Flow chart of biomarker classifier validation. Flow chart showing the samples used for classifier generation and the validation results. (c) Heat map showing hierarchical clustering of 18 infant samples (9 bacterially infected, 6 control, 3 virally infected) based on the 50 probes that were in common between the classifier gene set and the Affymetrix U219 platform. Hierarchical clustering was based on Euclidean distance. Control, blue; bacterial infected, red; viral infected, black. Classification of bacterial infection is indicated (0=non-infected, 1=infected). (d) Comparison of microarray-based classifier and expert assessment for classification of samples from patients with suspected infection. (Top) Comparison of expert assessment, CD69/FCGR1A and the 52-gene classifier on samples scored ‘high’ and ‘low’ likelihood of infection by expert assessment. (Middle) 52-gene classifier prediction and expert assessment of suspected sepsis cases (red=concordance of ‘infection’, blue=concordance of ‘control’, dark grey=discordance of microarray classifier and expert assessment). (Bottom left) Comparison of CD69/FCGR1A and 52-gene classifier of samples scored ‘medium’ likelihood of infection by expert assessment. Classification of bacterial infection is indicated (0=non-infected (pale blue), 1=infected (pink)). (Bottom right) Sensitivity, specificity and accuracy of CD69/FCGR1A and the 52-gene classifier against expert classification for suspected samples fromdtop. A heat map showing the 30 infant samples of suspected infection based on the 46 probes that were in common between the classifier gene set and the CodeLink platform is shown inSupplementary Fig. 7. (e) Bar plots showing clinical criteria in suspected infection cases as judged by the 52-gene classifier and expert assessment. Days on antibiotics and neutrophil counts are shown for samples based on classification of control (pale blue) and bacterial infection (pink) showing median and standard error of the median. Days on antibiotics, classifier prediction: infected:n=15 (excluding 2 missing values); control:n=12 (excluding 1 missing value). Days on antibiotics, expert assessment: infected:n=5 (excluding 1 missing value); control:n=14 (excluding 1 missing value). Neutrophil count, classifier prediction: infected,n=17; control,n=13. Neutrophil count, expert assessment: infected:n=6; control:n=15. Figure 7a shows the average LOOCV error rate over 100 replications as a performance measure with biomarkers listed sequentially. When the number of genes included was 19 or more the error rate was consistently 0% for all four machine-learning methods, thus confirming internal consistency of the selected markers as a classifier. Pleasingly, this number of genes is in excellent agreement with the computed optimal number of biomarkers ( n =24) from our previous in silico simulation studies [19] . For all subsequent testing, we proceeded with the ROC-based classifier [39] , as this does not require any tuning of parameters and simplifies classification to a univariate decision that can easily be applied to independent data. An analysis of the individual pathways using the ROC-based classifier provided an accuracy of 84% for innate markers, 65% for the adaptive markers and 74% with the metabolic markers; whereas all three pathway markers combined gave an enhanced accuracy of 98% (sensitivity=100%, specificity=97%). Hence, combination of the three pathways provides an optimally robust classifier. Figure 7: Validation of the 52-gene dual-network classifier. ( a ) Members of the network as a classifier of neonatal infection using leave-one-out cross-validation analysis using four independent machine-learning algorithms (red circle, random forest; green triangle, support vector machines; blue+, K nearest neighbour and black x, receiver operator characteristics). ( b ) Flow chart of biomarker classifier validation. Flow chart showing the samples used for classifier generation and the validation results. ( c ) Heat map showing hierarchical clustering of 18 infant samples (9 bacterially infected, 6 control, 3 virally infected) based on the 50 probes that were in common between the classifier gene set and the Affymetrix U219 platform. Hierarchical clustering was based on Euclidean distance. Control, blue; bacterial infected, red; viral infected, black. Classification of bacterial infection is indicated (0=non-infected, 1=infected). ( d ) Comparison of microarray-based classifier and expert assessment for classification of samples from patients with suspected infection. (Top) Comparison of expert assessment, CD69/FCGR1A and the 52-gene classifier on samples scored ‘high’ and ‘low’ likelihood of infection by expert assessment. (Middle) 52-gene classifier prediction and expert assessment of suspected sepsis cases (red=concordance of ‘infection’, blue=concordance of ‘control’, dark grey=discordance of microarray classifier and expert assessment). (Bottom left) Comparison of CD69/FCGR1A and 52-gene classifier of samples scored ‘medium’ likelihood of infection by expert assessment. Classification of bacterial infection is indicated (0=non-infected (pale blue), 1=infected (pink)). (Bottom right) Sensitivity, specificity and accuracy of CD69/FCGR1A and the 52-gene classifier against expert classification for suspected samples from d top. A heat map showing the 30 infant samples of suspected infection based on the 46 probes that were in common between the classifier gene set and the CodeLink platform is shown in Supplementary Fig. 7 . ( e ) Bar plots showing clinical criteria in suspected infection cases as judged by the 52-gene classifier and expert assessment. Days on antibiotics and neutrophil counts are shown for samples based on classification of control (pale blue) and bacterial infection (pink) showing median and standard error of the median. Days on antibiotics, classifier prediction: infected: n =15 (excluding 2 missing values); control: n =12 (excluding 1 missing value). Days on antibiotics, expert assessment: infected: n =5 (excluding 1 missing value); control: n =14 (excluding 1 missing value). Neutrophil count, classifier prediction: infected, n =17; control, n =13. Neutrophil count, expert assessment: infected: n =6; control: n =15. Full size image Next, replication and validation of the classifier on different microarray platforms and patient samples that were not part of the original gene selection process was performed ( Fig. 7b and Supplementary Fig. 11 ). In our platform test set, we used 42 of the training-set samples (18 infected, 24 controls) for 48 (matched) genes with a completely different microarray platform. A ROC classifier when applied to this platform correctly assigned 100% of samples to control or bacterially infected groups (sensitivity=100%, specificity=100%). In our validation test set, we used a completely new independent set of 26 samples (16 infected and 10 controls) that were analysed on three different microarray platforms. ROC classification based on the training set when applied to the new validation test set correctly assigned 100% of samples to control or bacterially infected groups with sensitivity=100% and a specificity=100% ( Supplementary Dataset 3 ). Notably, a further three virally infected samples classified as control and align with control samples in hierarchical clustering ( Fig. 7c ). These results are in agreement with the CMV-infected case shown in Fig. 1 that is also not recognized by the dual-network and also clustered with the controls and not bacterially infected samples. We compared the outcome of the 52-gene dual-network with recently published host protein biomarkers (CD69 and FCGR1A) of neonatal sepsis that have been reported to have 100% sensitivity and 22–44% specificity [16] . It is worth noting that FCGR1A is a member of the dual-network classifier. For this purpose, we tested whether expression levels of CD69 and FCGR1A (CD64) would sufficiently predict infection on the training set. We trained the ROC-based classifier on these two genes with the 62-sample training set and used LOOCV to assess its accuracy within the same set. The LOOCV analysis of these markers at the RNA level developed 74% sensitivity with 91% specificity with an overall accuracy of 84%. Although these results show the potential use of these markers, they clearly exhibit sensitivity values less than specificity and have reduced accuracy in comparison with the 52-gene dual-network classifier that is more robust against sample-to-sample variation of individual genes. The most pressing clinical need is to identify bacterial infection in individuals that are suspected to have infection at the first time of symptoms developing, who subsequently have negative bacterial cultures. To investigate this, we selected a completely new group of 30 patients who were suspected of being infected at the time of sample collection but who had blood culture-negative test results. The 52-gene ROC classifier applied to this suspected infected test set assigned 17 of the 30 patient samples to the bacterially infected group ( Fig. 7d ). Subsequent expert assessment based on clinical criteria indicated 6 infected and 15 non-infected samples ( Fig. 7d top) with 9 samples where a clinical categorization could not be confidently made ( Fig. 7d bottom left). Concordance between classifier prediction and expert opinion for the infected and non-infected was moderate (Cohen’s kappa k =0.24, in relation to the empirically achievable k =0.46; Fig. 7d middle) and comparison of classifier predicted infection with expert assessment showed good agreement with statistically significant differences in days on antibiotics and neutrophil count between classified control and infected suspected samples ( Fig. 7e ). For comparison, the predictions of the CD69+FCGR1A are shown in Fig. 7d top and bottom, and exhibits a very low concordance based on Cohen’s kappa test for the CD69/FCGR1A classifier versus expert assessment of k =0.05 out of an empirically possible k =0.40. In addition, using the Expert opinion as ‘gold-standard’, Fig. 7d bottom right shows the much reduced accuracy values for CD69/FCGR1A in contrast to the 52-gene classifier. These findings highlight the difficulty faced by clinicians in determining cases of blood culture-negative sepsis and strongly support the future clinical utility of the 52-gene classifier. We conclude that the 52-gene dual-network has excellent efficacy for predicting bacterial infection. 52-Gene dual-network is robust against gestational age In considering the demographic data, it is evident that there is a difference in mean corrected gestational age of infected and controls. Hence, it is important to be sure that gene expression levels of the 52-genes are not a reflection of differing maturity of the immune system. We therefore examined our classifier gene set by looking at gene expression within groups according to gestational age. Notably, we find there is no statistical difference in gene expression of the 52-gene dual-network between infants of differing gestational ages ( Supplementary Table 2 ). Therefore, in this study group, the dual-network trait is robust against variation across gestational ages. It is also noteworthy that although a statistically significant increase in neutrophils is detected ( Fig. 3d ), the dual-network is reliable in stratifying infected infants who had neutropenia and also fails to detect viral-infected cases. To test for a dependence on gestational age for any of the 824 genes altered in sepsis, we applied a linear model to the sepsis samples of the training set for each gene by regressing the gestational age as a continuous variable. No statistically significant age-dependent effects were found after false discovery rate correction. Hence, any confounding issue with gestational age is statistically non-discernable for sepsis cases. As this analysis does not rule out nonlinear association, we repeated this analysis with cubic and quadratic regressive fits for gestational age, and found no significant associations. Thus, although we cannot absolutely rule out a confounding factor associated with gestational age, our analysis indicates that the alterations in sepsis cases is due to host immune response to infection. Here, we report the underlying in vivo molecular phenotype of microbiologically confirmed neonatal sepsis. Strikingly, we find a highly exacerbated and unbalanced homeostatic systemic innate immune and metabolic response, which is accompanied by a reduced lymphoid involvement. The strength and magnitude of these changes show the remarkable ability of the neonate to recognize and acutely mount a vigorous but highly focused response. The response is not a ‘storm’ but instead exhibits an altered set-point in the regulatory communication between innate and adaptive immune cells. At the patient level, an individualized assortment of functionally related modules of expressed genes is present. Despite this heterogeneity, a more consistent response of a 52-gene dual-network consisting of three pathways, innate, metabolic and adaptive immune pathways, is developed and can identify with high accuracy bacterially infected, but not in virally infected, cases examined. It is noteworthy that necrotizing enterocolitis samples classified positive for infection ( Supplementary Data set 3 ), supporting the case for a high level of specificity in the molecular systemic response to infection. For future translational work, more sensitive and specific results would enable empirical antibiotics to be avoided in all but the most critically ill newborns. This is critically important given concerns that empirical antibiotics may increase the risks of developing necrotizing enterocolitis and mortality in premature infants [40] . The scale of changes detected in neonates is vastly different from those recorded in adults, although at an individual gene or protein analytic level some of our findings are consistent with those of studies carried out in older populations [41] . Elevated TLRs have been observed in adult pre-sepsis [42] and in children with septic shock [43] . Downregulation of T-cell signalling, antigen processing and reduced HLA II expression [43] , [44] , [45] , [46] has also been described previously in adult and paediatric sepsis and in fetal inflammatory response syndrome [10] . However, there are also clear differences, for instance, IFNγ -IL12 axis, while detectable is not differentially activated as observed in older population groups [11] and agrees with previous studies on the role of IL12 in neonatal sepsis [47] . Also notable are elevated levels of myeloid-derived suppressor cell markers that may affect the set point in the regulatory cross talk with the lymphoid compartment. Other key homeostatic regulatory mediators include FFAR2 that is regulated by short-chain fatty acids derived from the gut microbiota that mediate an anti-inflammatory role in immune cell function as well as lipid energy metabolism. Altogether, these responses support the notion of alterations in the homeostatic control mediated by the regulatory interplay between the microbiota, innate and adaptive immunity [24] . The set point for immune control is extended to the regulation in co-stimulatory signalling between antigen-presenting cell and T cells, and in neonatal sepsis we, find a highly focused inhibitory co-stimulatory response mediated through marked upregulation of, especially, CD85 receptors that have inhibitory functions. Concomitantly, a broad array of cell intrinsic immune repressors are also significantly upregulated, including IL1R2, ILRN, A20, IκBα, (NFKB1A) TOLLIP, IRAKM, TRAIL-R3, TRAFD1, SOCS1 and SOCS3. These observations provide new insight into the homeostatic control mechanisms involved in governing the immune response in sepsis. The immune homeostatic set point mechanistically determines the level at which the innate immune system activates the adaptive response. Thus, in neonatal sepsis, we propose that a heightened homeostatic set point culminates in a regulatory suppressed response. Patient recruitment and power calculations The study was conducted in the Neonatal Unit, Royal Infirmary of Edinburgh, and the Division of Pathway Medicine, University of Edinburgh. Infants having blood cultures taken to investigate suspected infection ( Supplementary Table 3b ) and ‘well’ control infants having blood taken for other clinical reasons ( Supplementary Table 3c ) were studied. A more extensive list of clinical criteria assessed for all samples used in the study are provided in Supplementary Data set 4 . Five infants had samples included from more than one episode of infection. After parent consent, we obtained blood samples at the time of first clinical signs of suspected infection with an additional 0·5–1 ml of whole blood for expression profiling collected alongside the ‘gold-standard’ microbiological blood culture. Samples taken from patients with suspected clinical infection that proved to have microbiological evidence of infection from a usually sterile body site were identified and formed the infected group. Full clinical assessment for early and late symptoms and signs of sepsis followed criteria for neonatal sepsis taken from data as detailed in Supplementary Data set 4 , with the blood culture test used as the ‘gold standard’ for diagnosis of sepsis. For patient samples with coagulase-negative staphylococcus full clinical assessment was conducted independently by two clinicians (CLS and BJS/JO) and clinical evidence supporting or refuting inclusion was reviewed. The neonatal unit uses the definitions of the Vermont Oxford Network for infection surveillance [48] and associated clinical deterioration, repeat isolates and deranged blood counts were also examined. Samples were only included as positive if both clinicians agreed that infection was present. This was conducted blind to the results of any RNA expression profile data. For power calculations, samples were obtained from 30 infants at 9 months of age, before vaccination. To meet with laboratory regulations, samples that could be considered ‘high risk’ were excluded. Infants were not included in the study if the mother was known to be positive for hepatitis B, HIV or hepatitis C viruses. In cases where the mother was known to have a history of drug misuse and had not had antenatal screening for blood-borne viruses, the infants were also excluded. Other exclusion criteria were infants who did not require clinical blood samples and infants for whom extra blood sampling might be of particular risk, for example, infants with an underlying disorder causing anaemia. For RNA isolation, blood was immediately injected into a PAXgene blood RNA tube. Frozen samples were subjected to RNA extraction and microarray analysis performed. Before embarking on this study, we performed a power calculation using the Illumina chip platform, on an independent set of 30 infant samples ( Supplementary Fig. 8 ). This shows that the study design has 90% power to detect a twofold change in expression with an α of 1% (false discovery rate (FDR) corrected), for more than 99% of 35,177 gene probes present on the array. RNA was extracted using a protocol validated for use in small volume neonatal blood samples [18] . Patient sample analysis workflow and study design The patient demographics, microbial organisms isolated and reasons for blood sampling in controls for all patient sets are shown in Supplementary Table 3 . All samples were processed for genome-wide transcriptional analysis using microarrays. On the basis of power calculations ( Supplementary Fig. 8 ), sample size of approximately 25 for each group has ≥90% power to detect twofold changes in expression level of 99% of probes on the microarray. A schematic of patient recruitment and sample processing workflow for the 285 samples processed for the main study and validation arm is shown in Supplementary Fig. 9 . For the computational and statistical pathway biology aspects of this study, a summary of data analysis workflow and associated figures are provided in Supplementary Fig. 10 . The main study arm primarily used RNA profiling data using the Illumina HT12 platform from 27 patient samples with a confirmed blood culture-positive test for sepsis (bacterial infected cases), 1 cytomegalovirus (CMV)-infected case and 35 matched controls. Samples from these cases (not including the viral infected case) are referred to as the ‘training set’ in this study. For assessing reproducibility with a different assay platform, we examined a subset of 42 of these samples using the CodeLink gene expression platform (comprising 18 bacterial infected and 24 control samples) named in this study as ‘platform test set’. Subsequently, for independent clinical evaluation, the 52-gene set classifier was applied to a further 29 new and independent samples (comprising 16 bacterial infected, 3 viral infected and 10 control samples) named in this study as ‘validation test set’. CodeLink data used in the platform and validation test sets developed a variable but acceptable maximal density for approximately 50% of chips analysed. Finally, a set of 30 new samples collected upon suspicion of infection but with negative blood culture were analysed, named in this study as ‘suspected infected test set’. A detailed summary of the workflow for the training and testing of the 52-gene set classifier of sepsis in neonates is shown in Supplementary Fig. 11 . Statistical analysis High-quality RNA from infected and control infants was hybridized onto Illumina Human Whole-Genome Expression BeadChip HT12v3 microarrays comprising 48,802 features (human gene probes). Microarray quality analysis used the arrayQualityMetrics package in Bioconductor [49] and a gender check was performed using Y-chromosome-specific loci. Using the ‘lumi’ Bioconductor package, raw data from 63 samples were transformed using a variance stabilizing transformation before robust spline normalization to remove systematic between-sample variation. Microarray features that were not detected, using detectionCall on any of the arrays, were removed from analysis and the remaining 23,342 features were used for subsequent statistical analysis. Data were statistically examined to assess gestational age as a confounding factor. Within each sample group (control, infected), samples were age classified into bins based on the 33 and 66% corrected gestational age quantile values, yielding three age groupings. Comparison of normalized data between groups utilized linear modelling of the log 2 scale expression values between groups and subsequent empirical Bayesian approaches to moderate the test statistic by pooling variance information from multiple genes. This included vertical P -value adjustment for multiple testing (Benjamini–Hochberg) to control for false discovery rate using the Bioconductor package ‘limma’ [50] . Statistically significant differentially expressed genes were examined further: heat maps and line graphs with hierarchical clustering by Euclidean distance were examined using Partek Genomics Suite v6·5, and visualization of networks of genes looking for patient-specific responses using BioLayout Express 3D [37] . Unsupervised clustering of patient samples was carried out: probes with coefficient of variation greater than 0.1 were used (10,206) and hierarchical clustering was based on Euclidean distance. For purposes of classification, we refer to the 62 Illumina-hybridized samples with the selected subset of 52 genes as ‘training set’. We employ multiple types of classification test sets, which are defined as follows ( Supplementary Fig. 9 ). In addition to the Illumina microarray analysis, we examined a subset of 42 of these samples (18 infected, 24 controls) using CodeLink Whole Human Genome arrays, referred to as ‘platform test set’. Subsequently, the classifier was applied to a further 26 new and independent samples (16 bacterially infected samples from 15 infants and 10 control samples), which were run on CodeLink (7 infected and 3 control), Affymetrix HG-U133 (two infected, three control) or Affymetrix Human Genome U219 (9 infected and 6 control) arrays. These are collectively referred to as ‘validation test set’. We also assess the performance of our classifier on 30 independent samples with suspected but initially unconfirmed infection (CodeLink arrays) and refer to this as ‘suspected infected test set’. Use of the term ‘classifier’ refers to the classification algorithm and its trained state based on our set of 52 biomarkers. In discussion of the set of 52 biomarkers themselves, we refer to these as ‘classifier gene set’ or ‘52-gene classifier’. before training and testing the ROC-based classifier on the training and test sets, the original log 2 expression values for the 52-gene set were scaled to mean=0 and standard deviation=1 (that is, z-transformation per sample). The data scaling allows for prediction of biological samples on a separate microarray platform from that used in training the classifier. This ROC-based classification algorithm does not require any parameter optimization or tuning because its only parameter is the number of predictor genes to be used, which is in this case pre-determined as the number of genes suggested as predictors through prior analysis. The same scaling procedure (independently applied to this small subset of genes) was used to test a previously published gene set (CD69, FCGR1A) for performance on our training set of 62 Illumina microarray samples. Network and pathway analysis Computational network-based approaches were used to examine relationships in the data using correlation of gene expression and biological relationships. IPA ( http://www.ingenuity.com ), DAVID [51] and a manually curated data set of human gene interactions in InnateDB ( http://www.innatedb.com ) [22] were used to examine biological network relationships and association with known pathways, for example, Kyoto Encyclopedia of Genes and Genomes [52] . The InnateDB network was analysed using Cytoscape 2.6.3 (ref. 53 ) and the cytoHubba plugin [54] to investigate a variety of properties of a network including the identification of network hubs and bottlenecks, which may represent the key regulatory nodes in the network. The network was also analysed to identify ‘active sub-networks’ using the jActiveModules [23] plugin to identify densely connected differentially expressed sub-networks. Cellular localizations of network components were visualized using cytoscape and the Cerebral v.2 (ref. 55 ) plugin. The contribution of specific blood cell subsets was examined by categorizing responses according to cell type using cell-specific gene markers described by Abbas and colleagues [21] . Pathway analyses were carried out step-wise using a pathway biology approach, becoming more focused until a defined sub-network of 52 differentially expressed genes was identified. The selected genes had adjusted P values of ≤10 −5 , fold changes of ≥4 and were highly connected in terms of biological pathways and networks. Classifier analysis These 52 genes were then assessed for prediction precision in a LOOCV error modelling using four different classification methods: random forests, support vector machines, K nearest neighbour and ROC-based classification. LOOCV was repeated 100 times for each set of selected genes following a random ordering of the data at each replication to minimize variability of the error estimates. For independent technical validation of RNA expression levels of the classifier gene set outside the neonatal sample set used for feature selection, a subset of samples run on CodeLink Human Whole-Genome microarrays was examined (platform test set). The subset was chosen only by virtue of being previously run on CodeLink. ROC classification [39] was used to repeat the internal cross-validation on this subset using the markers that were present on both arrays and then using the trained classifier to predict the CodeLink samples. For further validation, a new sample set of 16 bacterially infected and 10 control samples (not previously used for feature selection or other analyses, but obtained in the same study setting with the same sample collection protocol) run on CodeLink, Affymetrix Human Genome HG-U133 Plus 2·0 or Affymetrix Human Genome U219 arrays had the ROC-based classifier applied (validation test set). All classification analyses were performed with R [56] , classification error in relation to gene set size was performed with the R package ‘optBiomarker’ [19] and ROC-based classification uses the R package ‘rocc’ [39] . Study approval Written informed consent was obtained from parents of all enrolled infants in accordance with approval granted by the Lothian Research Ethics Committee for blood samples for RNA isolation obtained at the first time of clinical signs of suspected sepsis (reference 05/s1103/3). Samples used in power calculations were collected with the approval of the Gambia Government/MRC Laboratories Joint Ethics Committee and London School of Tropical Medicine ethics committee (reference SCC1085, L2008.63). How to cite this article: Smith, C. L. et al . Identification of a human neonatal immune-metabolic network associated with bacterial infection. Nat. Commun. 5:4649 doi: 10.1038/ncomms5649 (2014). Accession codes: Microarray data has been deposited in Gene Expression Omnibus with accession code GSE25504 .